Long non-coding RNA-mediated transcriptional interference of a permease gene confers drug tolerance in fission yeast Most long non-coding RNAs (lncRNAs) encoded by eukaryotic genomes remain uncharacterized. Here we focus on a set of intergenic lncRNAs in fission yeast. Deleting one of these lncRNAs exhibited a clear phenotype: drug sensitivity. Detailed analyses of the affected locus revealed that transcription of the nc-tgp1 lncRNA regulates drug tolerance by repressing the adjacent phosphate-responsive permease gene transporter for glycerophosphodiester 1 ( tgp1 + ). We demonstrate that the act of transcribing nc-tgp1 over the tgp1 + promoter increases nucleosome density, prevents transcription factor access and thus represses tgp1 + without the need for RNA interference or heterochromatin components. We therefore conclude that tgp1 + is regulated by transcriptional interference. Accordingly, decreased nc-tgp1 transcription permits tgp1 + expression upon phosphate starvation. Furthermore, nc-tgp1 loss induces tgp1 + even in repressive conditions. Notably, drug sensitivity results directly from tgp1 + expression in the absence of the nc-tgp1 RNA. Thus, transcription of an lncRNA governs drug tolerance in fission yeast. Eukaryotic genomes are pervasively transcribed. Frequently this transcription generates long non-coding RNAs (lncRNAs), which may be transcribed antisense to protein-coding genes, from within introns, or from intergenic regions of the genome. RNA polymerase II (RNAPII) is responsible for generating both messenger RNAs (mRNAs) and lncRNAs [1] . As with mRNAs, many lncRNAs are processed (that is, capped, spliced, polyadenylated), however, in contrast to protein-coding mRNAs, lncRNAs are predominantly nuclear and many are rapidly degraded by the exosome [2] , the major cellular 3′→5′ RNA degradation machinery [3] . Consequently, the majority of lncRNAs exhibit low steady-state levels compared with mRNAs. This instability coupled with their general lack of primary sequence conservation has lead to the suggestion that many lncRNAs might simply result from spurious, inconsequential ‘transcriptional noise’ [4] . Nonetheless, accumulating evidence indicates that an increasing number of lncRNAs act to regulate gene expression [2] , [5] . The mere act of lncRNA transcription, including accompanying chromatin modifications and resulting changes in nucleosome density [6] , can have a profound impact on neighbouring gene expression. In the simplest scenario, lncRNA expression can provide an environment that is either suitable or unsuitable for transcription factor binding. For example, cascading lncRNA transcription upstream of the fission yeast Schizosaccharomyces pombe fbp1 + gene is required to induce fpb1 + expression following glucose starvation [7] . In addition, in a process termed ‘transcriptional interference’, serine-mediated repression of the budding yeast Saccharomyces cerevisiae SER3 gene is brought about by lncRNA transcription into the gene promoter, which increases nucleosome density and prevents transcription factor access [8] , [9] , [10] . These examples illustrate the positive and negative influence that lncRNA transcription can exert on gene regulation in response to environmental changes. lncRNAs can also be processed into smaller regulatory RNAs (for example, short interfering RNA) [11] . In S. pombe , lncRNAs transcribed from centromeric outer repeats are processed by Dicer (Dcr1) into short interfering RNAs, which target the Clr4 H3K9 methyltransferase via Ago1 (within the RNA-induced transcriptional silencing complex) to establish repressive heterochromatin through the methylation of lysine 9 on histone H3 (refs 12 , 13 , 14 , 15 ). In addition, lncRNAs may directly associate with and recruit factors that alter chromatin status, in cis or in trans , silencing genes or behaving as enhancers [16] , [17] . For example, lncRNAs aid the response of S. cerevisiae cells to specific changes in nutrient availability by recruiting chromatin-modifying complexes (for example, histone deacetylases) to dynamically regulate several genes [18] , [19] , [20] . Related mechanisms have since been reported in multicellular eukaryotes [21] , [22] . Recent analyses also suggest that patches of transient heterochromatin can form under particular conditions at specific euchromatic loci in S. pombe [23] , [24] , [25] . This mechanism involves the RNA-binding protein Mmi1, which recruits the RNA-surveillance machinery to specific determinant of selective removal (DSR) motifs in target transcripts, leading to their exosome-mediated degradation [26] . Mmi1 and its associated factor Red1 are reported to also recruit chromatin-modifying activities via nascent mRNA and lncRNA targets to deposit H3K9 methylation (H3K9me2) at these locations [23] , [25] , [27] , [28] . It is therefore evident that lncRNAs employ a variety of mechanisms to regulate gene expression. Despite rapid advances in lncRNA identification, only a small number have been characterized in detail. A clear challenge in assigning function has been a lack of lncRNA sequence conservation between even the most closely related species [29] . However, the order of genes flanking the transcription units that encode lncRNAs can be preserved through evolution [30] (that is, synteny) and provides another criterion by which we can identify potential functionally conserved lncRNAs whose primary sequences might have diverged too much so as not to retain detectable homology. Only a few of the ~500 annotated intergenic lncRNAs in S. pombe are conserved at the sequence level in three divergent Schizosaccharomyces species, although many retain synteny with flanking genes in at least one other species [31] . We identified eight discrete intergenic lncRNAs that exhibit synteny in at least three of the four Schizosaccharomyces species. Deletion of one of these loci (SPNCRNA.1343 or ncRNA.1343 for short) exhibited a drug-sensitivity phenotype. We demonstrate that ncRNA.1343 encodes a bidirectional lncRNA promoter and that its deletion causes loss of expression of the divergent unstable transcript nc-tgp1 . Our analyses reveal that nc-tgp1 is targeted for Mmi1-directed exosome degradation and is required to repress a downstream phosphate-responsive gene (SPBC1271.09 designated transporter for glycerophosphodiester 1 (tgp1 + )). However, rather than involving transient heterochromatin formation as a result of targeted RNA degradation, the regulation of tgp1 + by the nc-tgp1 RNA appears to be mediated by transcriptional interference. Most importantly, tolerance of S. pombe to a broad spectrum of compounds relies on the regulation of tgp1 + by nc-tgp1 . Deletion of SPNCRNA.1343 causes drug hypersensitivity The S. pombe genome is predicted to encode ~500 intergenic lncRNAs [32] . Although few of these lncRNAs exhibit detectable sequence conservation, ~100 are conserved in synteny with putative lncRNA orthologues in at least one of the three other known Schizosaccharomyces species [31] . For example, the functionally characterized telomerase RNA ( ter1 + /SPNCRNA.214) is syntenic despite its lack of sequence conservation (see Supplementary Fig. 1a ). To identify other potential functionally conserved lncRNAs, we selected eight lncRNAs, including ter1 + as a control, where surrounding gene order is retained in S. pombe and at least two other Schizosaccharomyces species. Each lncRNA gene was deleted by replacement with a loxP-flanked ura4 + marker ( Supplementary Fig. 1b ). Apart from ter1Δ , the selected lncRNAs were not essential for normal cell growth ( Supplementary Figs 1c and 2 ). However, since many characterized lncRNAs regulate gene expression in response to environmental changes and stress [33] , we tested the growth of these lncRNA deletion strains in response to the following stresses: temperature, the microtubule destabilizing drug thiabendazole (TBZ), DNA synthesis inhibitor hydroxyurea (HU), ultraviolet-induced DNA damage, H 2 O 2 -induced oxidative stress and caffeine, an inhibitor of cyclic AMP phosphodiesterase. Cells lacking SPNCRNA.1343 ( ncRNA.1343 for short) displayed a phenotype: hypersensitivity to TBZ, HU and caffeine but not to temperature extremities, ultraviolet-irradiation or oxidative stress ( Supplementary Fig. 1c and Supplementary Fig. 2 ). Drug sensitivity of 1343Δ cells is caused by tgp1 + induction lncRNAs can act in cis to regulate the expression of nearby genes [2] . To determine the cause of drug sensitivity in 1343Δ cells we examined the expression of genes flanking the locus by real-time quantitative reverse transcriptase-PCR (RT–qPCR) in wild-type cells, cells with ncRNA.1343 replaced by loxP-flanked ura4 + marker ( 1343Δ::ura4 + ) and cells with the ura4 + marker subsequently removed ( 1343Δ ; Fig. 1a ). SPBC1271.09 transcript levels increased >50-fold in both 1343Δ::ura4 + and 1343Δ cells ( Fig. 1b ), while the expression of other neighbouring genes was unaltered. SPBC1271.09 encodes a conserved glycerophosphodiester membrane transporter (designated as tgp1 + ) orthologous to the S. cerevisiae permease GIT1 . As with S. cerevisiae GIT1 , the tgp1 + gene is repressed when cells are grown in the presence of phosphate and induced upon phosphate starvation [34] , [35] . Northern analysis confirmed that tgp1 + was indeed highly expressed in 1343Δ cells but not wild-type cells, both grown in the presence of phosphate (repressed condition; Fig. 1c ). 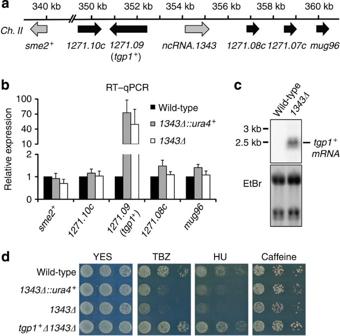Figure 1: Drug sensitivity followingncRNA.1343deletion is due to increasedtgp1+expression. (a) Schematic representation of genes flankingncRNA.1343. (b) RT–qPCR experiments measured transcript levels for nearby genes in wild-type cells and following replacement ofncRNA.1343withura4+(1343Δ::ura4+) or deletion (1343Δ). Error bars represent s.e.m. resulting from at least three independent replicates. (c) Northern analysis oftgp1+transcript levels in wild-type and1343Δcells grown in the presence of phosphate. (d) Serial dilutions of wild-type,1343Δ::ura4+,1343Δandtgp1Δ1343Δdouble mutant spotted on non-selective YES medium or in the presence of TBZ (20 μg ml−1), HU (10 mM) or caffeine (15 mM), respectively. Figure 1: Drug sensitivity following ncRNA.1343 deletion is due to increased tgp1 + expression. ( a ) Schematic representation of genes flanking ncRNA.1343 . ( b ) RT–qPCR experiments measured transcript levels for nearby genes in wild-type cells and following replacement of ncRNA.1343 with ura4 + ( 1343Δ::ura4 + ) or deletion ( 1343Δ ). Error bars represent s.e.m. resulting from at least three independent replicates. ( c ) Northern analysis of tgp1 + transcript levels in wild-type and 1343Δ cells grown in the presence of phosphate. ( d ) Serial dilutions of wild-type, 1343Δ::ura4 + , 1343Δ and tgp1Δ1343Δ double mutant spotted on non-selective YES medium or in the presence of TBZ (20 μg ml −1 ), HU (10 mM) or caffeine (15 mM), respectively. Full size image To determine whether the drug sensitivity of 1343Δ cells is a direct result of increased tgp1 + expression, the tgp1 + gene was deleted from 1343Δ cells ( tgp1Δ1343Δ ). This manipulation restored TBZ, HU and caffeine tolerance to levels comparable with wild-type cells ( Fig. 1d ). We conclude that increased tgp1 + expression is directly responsible for the drug-sensitivity phenotype of cells lacking ncRNA.1343 . Bidirectional lncRNA promoter upstream of tgp1 + Previous RNA-seq analysis indicates that an lncRNA is transcribed in the sense orientation upstream of tgp1 + (refs 27 , 31 ). We identified two divergent transcriptional start sites arising within ncRNA.1343 : one lncRNA transcribed towards the tgp1 + gene ( nc-tgp1 ) and the other in the opposite orientation ( nc-1343 ; Fig. 2a ; Supplementary Fig. 3 ). lacZ reporter assays demonstrate that the bidirectional promoter drives greater levels of transcription in the nc-tgp1 direction ( Supplementary Fig. 3 ). This finding is consistent with Rpb1 Chromatin Immunoprecipitation (ChIP) analysis showing that RNAPII is enriched over the nc-tgp1 transcription unit, while much lower RNAPII levels are detected on nc-1343 ( Fig. 2b ). 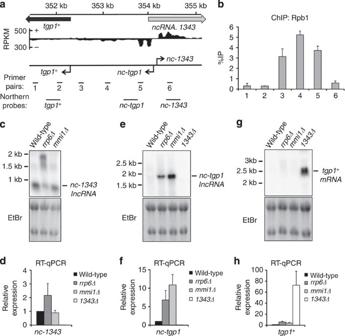Figure 2: Two distinct lncRNAs are transcribed from a bidirectional promoter upstream oftgp1+. (a) Previously published strand-specific RNA-Seq analysis (Rhindet al.,31) upstream of SPBC1271.09/tgp1+, represented as reads per kilobase per million (RPKM). Location of qPCR primer pairs and probes for Northern analysis are shown below. (b) Rbp1 ChIP–qPCR experiments performed in wild-type cells. (c,e,g) Northern analysis ofnc-1343,nc-tgp1andtgp1+transcript levels in wild-type,rrp6Δ,mmi1Δand1343Δ, respectively. (d,f,h) RT–qPCR experiments measurednc-1343,nc-tgp1andtgp1+transcript levels in wild-type,rrp6Δ,mmi1Δand1343Δ, respectively. Error bars represent s.e.m. resulting from at least three independent replicates. Figure 2: Two distinct lncRNAs are transcribed from a bidirectional promoter upstream of tgp1 + . ( a ) Previously published strand-specific RNA-Seq analysis (Rhind et al ., [31] ) upstream of SPBC1271.09/ tgp1 + , represented as reads per kilobase per million (RPKM). Location of qPCR primer pairs and probes for Northern analysis are shown below. ( b ) Rbp1 ChIP–qPCR experiments performed in wild-type cells. ( c , e , g ) Northern analysis of nc-1343 , nc-tgp1 and tgp1 + transcript levels in wild-type, rrp6Δ , mmi1Δ and 1343Δ , respectively. ( d , f , h ) RT–qPCR experiments measured nc-1343 , nc-tgp1 and tgp1 + transcript levels in wild-type, rrp6Δ , mmi1Δ and 1343Δ , respectively. Error bars represent s.e.m. resulting from at least three independent replicates. Full size image We next examined the regulation of the nc-1343 and nc-tgp1 transcripts produced from this bidirectional promoter. A ~0.9 kb transcript for nc-1343 was readily detected in wild-type cells. The size and levels of the nc-1343 transcript increased in exosome defective ( rrp6Δ ) cells, but not cells lacking Mmi1 or Red1 ( Fig. 2c,d ; Supplementary Fig. 4 ). The lncRNA corresponding to nc-tgp1 was previously detected in rrp6Δ and red1Δ cells [27] . We identified a consensus DSR motif for Mmi1 binding at position +820 nt within the nc-tgp1 transcript and RNA IP (RIP) experiments confirmed a direct interaction between Mmi1 and the nc-tgp1 RNA ( Supplementary Fig. 5 ). Northern analysis identified that an ~1.9 kb nc-tgp1 RNA accumulates in rrp6Δ , mmi1Δ and red1Δ , but not in wild-type cells ( Fig. 2e,f ; Supplementary Fig. 4 ). Interestingly, a recent study found that the repressive lncRNA transcribed upstream of the phosphate-responsive pho1 + gene in S. pombe also contains a DSR motif and is targeted by Mmi1 for exosome-mediated degradation [28] , indicating that a similar regulatory mechanism might control expression of tgp1 + and pho1 + . In sum, both nc-1343 and nc-tgp1 transcripts are processed by the exosome, but only nc-tgp1 is regulated by Mmi1-mediated recruitment of the nuclear exosome. A moderate increase in tgp1 + transcript levels has previously been reported in cells lacking Mmi1 (ref. 23 ). In agreement with this, we detected a similar increase (approximated four-fold) in tgp1 + transcript levels in mmi1Δ or exosome ( rrp6Δ or dis3-54 ) mutant cells by RT–qPCR, however, this increase is significantly less than the >50-fold upregulation of tgp1 + observed in 1343Δ cells ( Fig. 2g,h ; Supplementary Fig. 4 ). Moreover, we failed to detect the tgp1 + transcript in rrp6Δ or mmi1Δ cells by Northern analysis, indicating that tgp1 + is not induced in the absence of these factors. Thus, Mmi1-mediated exosome degradation is not the predominant mechanism involved in tgp1 + regulation. tgp1 + is repressed by the nc-tgp1 lncRNA The presence of the unstable nc-tgp1 RNA upstream of tgp1 + suggests that either nc-tgp1 , nc-1343 or both regulate tgp1 + expression. To test the involvement of these lncRNAs in tgp1 + regulation, a series of strategic genetic manipulations were performed ( Fig. 3a ). Truncations of nc-1343 (that is, AΔ and BΔ ) that retain its 5′ end did not result in the drug-sensitivity phenotype presented by 1343Δ cells ( Fig. 3b ) and, similarly, did not induce tgp1 + expression ( Fig. 3c ). This indicates that full-length nc-1343 is not required for tgp1 + repression. We next tested if nc-tgp1 is involved in repressing tgp1 + . Our analyses show that transcription of nc-tgp1 starts within the encoded ncRNA.1343 transcription unit ( Supplementary Fig. 3 ). Thus, deletion of the entire locus ( 1343Δ ) removes the nc-tgp1 promoter, and the 5′ end of its transcript, resulting in the observed loss of nc-tgp1 expression ( Figs 2f and 3c ). The AΔ and BΔ truncations of nc-1343 , which retain the nc-tgp1 promoter, do not affect nc-tgp1 transcription or relieve repression of tgp1 + . In contrast, interruption of the nc-tgp1 transcription unit by insertion of the ura4 + marker gene ( nc-tgp1:ura4 + ) prevented nc-tgp1 transcription, induced tgp1 + expression to levels observed in 1343Δ levels and increased sensitivity of these cells to TBZ, HU and caffeine ( Fig. 3b,c ). These analyses demonstrate that it is nc-tgp1 , not nc-1343 , that is critical for repressing tgp1 + in the presence of phosphate. 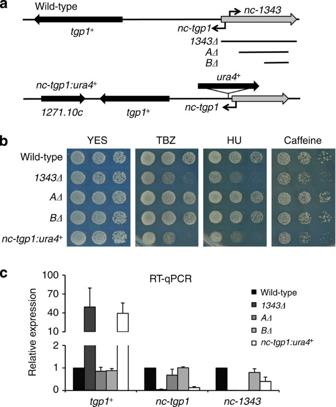Figure 3:nc-tgp1, notnc-1343, repressestgp1+to confer drug tolerance. (a) Schematic diagram indicating strategic manipulations of lncRNAs upstream oftgp1+including1343Δ, shorter deletions ofncRNA.1343(AΔandBΔ) andura4+integration within thenc-tgp1lncRNA locus (nc-tgp1:ura4+) in wild-type background. (b) Serial dilutions of wild-type,1343Δ, AΔ,BΔandnc-tgp1:ura4+were spotted on non-selective YES medium or in the presence of TBZ (20 μg ml−1), HU (10 mM) or caffeine (15 mM), respectively. (c) RT–qPCR experiments measuredtgp1+,nc-tgp1andnc-1343transcript levels in wild-type,1343Δ, AΔ,BΔandnc-tgp1:ura4+cells. Error bars represent s.e.m. resulting from three independent replicates. Figure 3: nc-tgp1 , not nc-1343 , represses tgp1 + to confer drug tolerance. ( a ) Schematic diagram indicating strategic manipulations of lncRNAs upstream of tgp1 + including 1343Δ , shorter deletions of ncRNA.1343 ( AΔ and BΔ ) and ura4+ integration within the nc-tgp1 lncRNA locus ( nc-tgp1:ura4 + ) in wild-type background. ( b ) Serial dilutions of wild-type, 1343Δ, AΔ , BΔ and nc-tgp1:ura4 + were spotted on non-selective YES medium or in the presence of TBZ (20 μg ml −1 ), HU (10 mM) or caffeine (15 mM), respectively. ( c ) RT–qPCR experiments measured tgp1 + , nc-tgp1 and nc-1343 transcript levels in wild-type, 1343Δ, AΔ , BΔ and nc-tgp1:ura4 + cells. Error bars represent s.e.m. resulting from three independent replicates. Full size image Phosphate starvation induces tgp1 + by repressing nc-tgp1 Upon phosphate starvation of fission yeast, several genes involved in the phosphate response are induced (including tgp1 + and pho1 + ) (ref. 35 ). To determine how the transcription of nc-tgp1 is altered in response to phosphate and how it might influence tgp1 + expression we assessed expression in phosphate-rich (+PO 4 ) and phosphate-deprived (−PO 4 ) conditions. As expected, the levels of tgp1 + and the pho1 + control increased upon phosphate starvation ( Fig. 4a,b ). In contrast, the levels of both nc-tgp1 and nc-1343 RNAs decreased significantly in the absence of phosphate ( Fig. 4a ; Supplementary Fig. 6 ). The observed reduction in nc-tgp1 levels is consistent with a situation whereby loss or reduction of nc-tgp1 transcription permits tgp1 + induction. In agreement with this, significantly less RNAPII associates with the nc-tgp1 transcription unit in both phosphate-starved wild-type cells and phosphate-replete 1343Δ cells, which do not transcribe nc-tgp1 ( Fig. 4c ). Therefore, preventing nc-tgp1 transcription, even in phosphate-rich medium, recapitulates the changes in RNAPII occupancy that normally accompany tgp1 + induction upon phosphate deprivation. 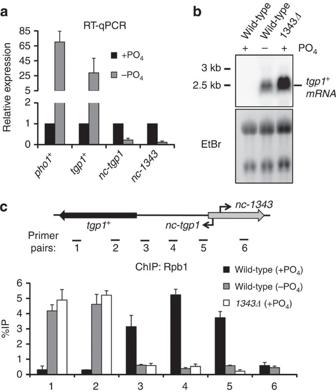Figure 4: Phosphate starvation inducestgp1+and reduces lncRNA transcription. (a) RT–qPCR experiments measuredtgp1+,nc-tgp1andnc-1343transcript levels in wild-type cells grown in phosphate-rich medium (+PO4) or in the absence of phosphate (−PO4).pho1+is a positive control for phosphate starvation. (b) Northern analysis oftgp1+in wild-type cells grown in the presence or absence of phosphate and1343Δgrown in the presence of phosphate. (c) Rbp1 ChIP–qPCR experiments performed in wild-type cells grown in the presence or absence of phosphate and1343Δgrown in the presence of phosphate. Error bars represent s.e.m. resulting from three independent replicates. Figure 4: Phosphate starvation induces tgp1 + and reduces lncRNA transcription. ( a ) RT–qPCR experiments measured tgp1 + , nc-tgp1 and nc-1343 transcript levels in wild-type cells grown in phosphate-rich medium (+PO 4 ) or in the absence of phosphate (−PO 4 ). pho1 + is a positive control for phosphate starvation. ( b ) Northern analysis of tgp1 + in wild-type cells grown in the presence or absence of phosphate and 1343Δ grown in the presence of phosphate. ( c ) Rbp1 ChIP–qPCR experiments performed in wild-type cells grown in the presence or absence of phosphate and 1343Δ grown in the presence of phosphate. Error bars represent s.e.m. resulting from three independent replicates. Full size image RNAi-directed heterochromatin does not repress tgp1 + Cells with defective exosome function ( rrp6Δ ) accumulate non-coding RNAs, some of which have been reported to attract Mmi1-dependent RNA elimination factors, along with RNA interference (RNAi) components and the Clr4 H3K9 methyltransferase, leading to the formation of transiently regulated HOODs (heterochromatin domains) [25] . The regions containing the tgp1 + and pho1 + genes are included in HOOD-17 and HOOD-24, respectively, and both form a region of Mmi1-directed transient heterochromatin in rrp6Δ cells [24] , [27] . The nc-tgp1 transcript is clearly regulated by Mmi1-directed exosome degradation ( Fig. 2e,f ), however, we do not detect methylated H3K9 (H3K9me2) over the tgp1 + , nc-tgp1 or nc-1343 genes within HOOD-17 in wild-type cells ( Fig. 5a ). Likewise, only very low levels of H3K9me2, slightly above background in cells lacking the H3K9 methyltransferase ( clr4Δ ), could be detected on the pho1 + gene and the upstream Mmi1-targeted lncRNA ( nc-pho1 ) within HOOD-24. Moreover, this low level of H3K9me2 did not drop appreciably upon induction of tgp1 + and pho1 + (−PO 4 ; Fig. 5a ). Equivalent background levels of H3K9me2 were detectable on another Mmi1-targeted lncRNA gene ( sme2 + ) and the highly expressed actin gene ( act1 + ). In contrast, H3K9me2 was ~100-fold enriched over the centromeric outer repeats ( dg ) in wild-type cells, but reduced to background in clr4Δ cells, indicating that H3K9-methylated chromatin had been efficiently immunoprecipitated. In addition, the transcript levels of tgp1 + , nc-tgp1 , nc-1343 , pho1 + and nc-pho1 were unaffected by loss of RNAi (for example, ago1Δ or dcr1Δ ) or heterochromatin components (for example, clr4Δ or swi6Δ ) ( Fig. 5b ; Supplementary Fig. 7a ). Nor were the kinetics of tgp1 + or pho1 + induction following phosphate starvation altered in cells lacking heterochromatin ( Supplementary Fig. 7b,c ). In contrast, nc-tgp1 , nc-pho1 and sme2 + RNA levels were clearly elevated in cells lacking Mmi1-mediated exosome degradation ( mmi1Δ and rrp6Δ ). Thus, although H3K9me2 accumulates at particular regions in rrp6Δ cells (for example, HOOD-17: tgp1 + and HOOD-24: pho1 + ), we conclude that RNAi and heterochromatin play no appreciable role in regulating these genes under normal physiologically repressive conditions or during their induction. 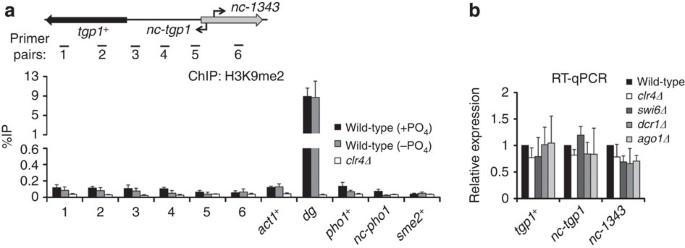Figure 5:tgp1+is not regulated by RNAi/heterochromatin. (a) H3K9me2 ChIP–qPCR experiments performed in the presence or absence of phosphate.clr4Δwas used as a negative control. The euchromatic actin gene (act1+) and centromericdgrepeats (dg) are positive and negative controls for heterochromatin.pho1+is a phosphate-regulated gene repressed bync-pho1, a lncRNA target of Mmi1.sme2+is another lncRNA target of Mmi1. H3K9me2 to bulk H3 ratio has not been presented due to background methyl H3K9 levels detected at these loci. (b) RT–qPCR experiments measuredtgp1+,nc-tgp1andnc-1343transcript levels in wild-type cells and cells lacking factors involved in heterochromatin formation and stability, respectively. Error bars represent s.e.m. resulting from at least three independent replicates. Figure 5: tgp1 + is not regulated by RNAi/heterochromatin. ( a ) H3K9me2 ChIP–qPCR experiments performed in the presence or absence of phosphate. clr4Δ was used as a negative control. The euchromatic actin gene ( act1 + ) and centromeric dg repeats ( dg ) are positive and negative controls for heterochromatin. pho1 + is a phosphate-regulated gene repressed by nc-pho1 , a lncRNA target of Mmi1. sme2 + is another lncRNA target of Mmi1. H3K9me2 to bulk H3 ratio has not been presented due to background methyl H3K9 levels detected at these loci. ( b ) RT–qPCR experiments measured tgp1 + , nc-tgp1 and nc-1343 transcript levels in wild-type cells and cells lacking factors involved in heterochromatin formation and stability, respectively. Error bars represent s.e.m. resulting from at least three independent replicates. Full size image nc-tgp1 prevents Pho7 transcription factor binding The above analyses indicate that nc-tgp1 is transcribed into the tgp1 + promoter and suggest that production of this upstream lncRNA represses tgp1 + expression. We therefore investigated if transcription of nc-tgp1 interferes with the induction mechanism of tgp1 + in response to phosphate starvation. The Pho7 transcription factor has previously been shown to engage phosphate-response gene promoters in phosphate-starved cells [35] , [36] . Our ChIP analyses confirmed that Pho7–green fluorescent protein (Pho7–GFP) accumulates on the pho1 + promoter in phosphate-depleted cells ( Supplementary Fig. 8 ). In addition, Pho7–GFP levels accumulate over the region upstream of tgp1 + when activated ( Fig. 6a ). However, in cells unable to transcribe nc-tgp1 ( 1343Δ ), higher levels of Pho7–GFP associate with the region upstream of tgp1 + even in repressive conditions (that is, +PO 4 ). We conclude that loss of nc-tgp1 expression due to phosphate starvation or by preventing production of this lncRNA (for example, 1343Δ ) allows Pho7 binding and subsequent tgp1 + induction. 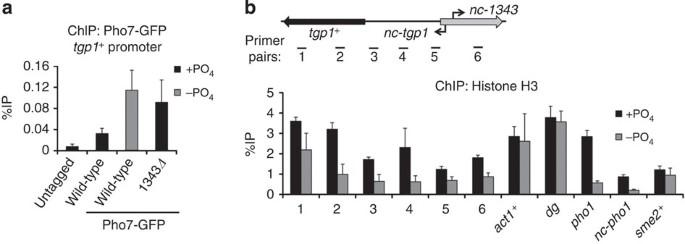Figure 6:nc-tgp1transcription prevents stable Pho7 binding and increases nucleosome density upstream oftgp1+. (a) GFP ChIP–qPCR experiments were performed in the presence or absence of phosphate in cells with C-terminally GFP-tagged Pho7. An untagged strain was used as a negative control. Primer pair #3 was used to detect Pho7 binding at thetgp1+promoter. (b) Nucleosome density was measured by histone H3 ChIP–qPCR experiments in wild-type cells grown in the presence or absence of phosphate. Error bars represent s.e.m. resulting from three independent replicates. Figure 6: nc-tgp1 transcription prevents stable Pho7 binding and increases nucleosome density upstream of tgp1 + . ( a ) GFP ChIP–qPCR experiments were performed in the presence or absence of phosphate in cells with C-terminally GFP-tagged Pho7. An untagged strain was used as a negative control. Primer pair #3 was used to detect Pho7 binding at the tgp1 + promoter. ( b ) Nucleosome density was measured by histone H3 ChIP–qPCR experiments in wild-type cells grown in the presence or absence of phosphate. Error bars represent s.e.m. resulting from three independent replicates. Full size image Active RNAPII promoters display reduced nucleosome density [37] . lncRNA transcription over promoters can increase nucleosome density and prevent gene induction [8] , [10] , [20] . We found that histone H3 levels were greater over the tgp1 + gene and upstream region when it is repressed (+PO 4 ) compared with when it is expressed (−PO 4 ; Fig. 6b ). In contrast, H3 levels over control loci ( act1 + , sme2 + and dg repeats) were unaffected by phosphate availability. Thus, upstream transcription appears to alter nucleosome density over the tgp1 + promoter and thereby occlude Pho7 binding. Likewise, a considerable drop in H3 levels was observed on the pho1 + gene and nc-pho1 lncRNA region upstream in phosphate-poor conditions, implying a similar mechanism may also operate to regulate the expression of pho1 + . We conclude that transcription of the upstream lncRNA inhibits expression of tgp1 + by a transcriptional interference mechanism that alters the chromatin landscape, preventing access to the key phosphate-responsive transcription factor Pho7. To directly test if transcriptional interference of tgp1 + by nc-tgp1 is responsible for tgp1 + repression, we replaced the nc-tgp1 promoter with the strong, thiamine-regulated nmt1 promoter ( nmt1-nc-tgp1 ) ( Fig. 7a ). Transcription of nc-tgp1 from the nmt1 promoter is rendered unresponsive to phosphate. Instead, nc-tgp1 is repressed or derepressed in the presence or absence of thiamine, respectively. When nc-tgp1 was transcribed from the nmt1 promoter, tgp1 + remained repressed regardless of phosphate availability ( Fig. 7b ). In contrast, repression of nmt1 -driven nc-tgp1 by thiamine resulted in the induction of tgp1 + expression in phosphate-rich media and consequently caused drug sensitivity ( Fig. 7b,c ). In addition, H3 levels over the region upstream of tgp1 + were high when nc-tgp1 was transcribed and reduced when nc-tgp1 was repressed by thiamine ( Fig. 7d ). Lastly, exogenous expression of full-length nc-tgp1 from a plasmid failed to repress tgp1 + , ruling out the possibility that nc-tgp1 operates in trans ( Supplementary Fig. 9 ). Collectively, these findings confirm that it is the transcription of nc-tgp1 over the tgp1 + promoter that alters nucleosome density to regulate tgp1 + induction (see Fig. 8 ) and, as a consequence, drug tolerance of fission yeast cells. 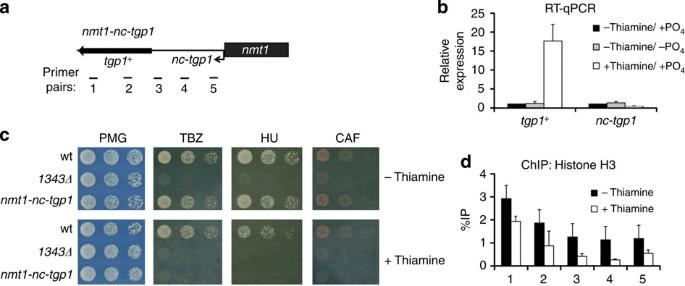Figure 7:nmt1controllednc-tgp1alters drug tolerance in response to thiamine. (a) Schematic diagram ofnc-tgp1under the control of the strong, thiamine-repressiblenmt1promoter. (b) RT–qPCR experiments measuredtgp1+andnc-tgp1levels in response to thiamine and phosphate availability usingnmt1-nc-tgp1cells. (c) Serial dilutions of wild-type,1343Δandnmt1-nc-tgp1cells were spotted on non-selective PMG medium or in the presence of TBZ, HU or caffeine, respectively, with or without thiamine as indicated. (d) H3 ChIP–qPCR experiments innmt1-nc-tgp1cells grown in the presence or absence of thiamine. Error bars represent s.e.m. resulting from three independent replicates. Figure 7: nmt1 controlled nc-tgp1 alters drug tolerance in response to thiamine. ( a ) Schematic diagram of nc-tgp1 under the control of the strong, thiamine-repressible nmt1 promoter. ( b ) RT–qPCR experiments measured tgp1 + and nc-tgp1 levels in response to thiamine and phosphate availability using nmt1-nc-tgp1 cells. ( c ) Serial dilutions of wild-type, 1343Δ and nmt1-nc-tgp1 cells were spotted on non-selective PMG medium or in the presence of TBZ, HU or caffeine, respectively, with or without thiamine as indicated. ( d ) H3 ChIP–qPCR experiments in nmt1-nc-tgp1 cells grown in the presence or absence of thiamine. Error bars represent s.e.m. resulting from three independent replicates. 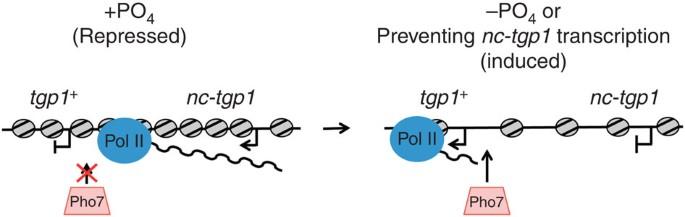Figure 8: Model for transcriptional interference attgp1+. The presence of phosphate induces transcription of an unstable lncRNA (nc-tgp1). lncRNA transcription increases nucleosome density, occludes Pho7 transcription factor binding and thus repressestgp1+expression.nc-tgp1transcription is reduced following phosphate starvation, decreasing nucleosome density, allowing Pho7 to stably engage thetgp1+promoter and inducetgp1+expression. Full size image Figure 8: Model for transcriptional interference at tgp1 + . The presence of phosphate induces transcription of an unstable lncRNA ( nc-tgp1 ). lncRNA transcription increases nucleosome density, occludes Pho7 transcription factor binding and thus represses tgp1 + expression. nc-tgp1 transcription is reduced following phosphate starvation, decreasing nucleosome density, allowing Pho7 to stably engage the tgp1 + promoter and induce tgp1 + expression. Full size image An increasing number of lncRNAs have been shown to tightly regulate eukaryotic gene expression following intra-/extra-cellular environment changes that require rapid, integrated responses at the level of transcription [2] . In S. pombe , for example, the balance of antisense lncRNAs and sense transcription controls various stress-response pathways [33] , [38] . However, little is known about the majority of S. pombe intergenic lncRNAs. Here we selected and deleted eight stable, discrete lncRNAs in S. pombe that show conserved synteny in at least two of the three other known Schizosaccharomyces species. Excluding the ter1 + control, only deletion of ncRNA.1343 exhibited a definitive phenotype: sensitivity to various compounds due to induction of a nearby phosphate-responsive permease gene ( tgp1 + ). Closer inspection revealed that the ncRNA.1343 promoter is bidirectional. Furthermore, transcription from this bidirectional promoter favours the production of a previously unannotated and unstable lncRNA ( nc-tgp1 ) towards the tgp1 + gene under repressive conditions. Recent studies in fission yeast have implicated lncRNAs in directing repression of specific genes by a mechanism involving transient RNAi-dependent heterochromatin formation [27] . For example, the Mmi1-targeted lncRNA upstream of pho1 + has recently been reported to recruit RNAi-directed heterochromatin to repress pho1 + in response to phosphate availability [28] . However, these findings differ from genome-wide H3K9me2 mapping which show that tgp1 + and pho1 + , both of which are regulated by upstream lncRNAs that are targeted for exosome-mediated degradation by Mmi1 ( Fig. 2 ; ref 28 ), only accumulate RNAi-directed H3K9me2 in mutants with defective RNA processing/degradation (for example, rrp6Δ ) and not in wild-type cells grown under repressive phosphate-rich conditions [24] . The significance of rrp6Δ -dependent heterochromatin at the tgp1 + and pho1 + genes is therefore unclear. Cells lacking Rrp6 accumulate aberrant RNAs and exhibit disrupted heterochromatin globally, including significantly decreased H3K9me2 over centromeric repeats [39] . Therefore caution must be exercised when interpreting the analyses of mutants with such severe defects in RNA processing/degradation. Importantly, we do not detect significant levels of H3K9me2 enrichment on the tgp1 + and pho1 + promoters/genes in wild-type cells under repressive (phosphate-rich) conditions. We cannot exclude the possibility that distinct assay conditions in a previous report allowed detection of low H3K9me2 levels on the pho1 + promoter when repressed [28] , however, the consequence of such H3K9me2 remains uncertain given that our analyses show that the expression of pho1 + or tgp1 + is unaffected by loss of RNAi/heterochromatin. We note that our findings are in agreement with previous expression profiling analyses, showing unaltered tgp1 + and pho1 + levels in S. pombe cells lacking RNAi/heterochromatin [40] . In contrast, transcripts arising from bone fide heterochromatin in centromeric outer repeats are clearly elevated when RNAi/heterochromatin is defective. Thus, our analyses indicate that the repression of both tgp1 + and pho1 + is unlikely to involve regulated heterochromatin in wild-type cells. Instead, we favour a model whereby tgp1 + and pho1 + are repressed by a transcriptional interference mechanism. Transcriptional interference is well-established in many systems. In the bacterium Escherichia coli , the gene encoding the clr transcriptional activator is repressed in response to nitrogen starvation by the act of lncRNA transcription from an alternate upstream promoter [41] . In the single celled eukaryote S. cerevisiae , which lacks RNAi and heterochromatin, transcription of the SRG1 lncRNA into the SER3 promoter, or heterologous promoters, was found to alter nucleosome density and interfere with transcription factor binding [8] , [9] , [10] . Similarly, in S. cerevisiae , non-coding transcription over the IME1 (ref. 20 ), GAL7 (ref. 42 ) and FLO11 (ref. 43 ) promoters prevent gene induction. Analogous mechanisms have also been reported in multicellular eukaryotes. For example, the Drosophila Ubx gene [44] , the human dihydrofolate reductase gene [45] and the imprinted Igf2r gene in mammals [46] are repressed independent of RNAi or transient heterochromatin formation by non-coding transcription into their respective promoters. These examples illustrate that transcriptional interference is a simple, conserved mechanism for modulating specific genes without requiring additional trans -acting regulatory factors. Our results are consistent with both nc-tgp1 and nc-pho1 mediating repression of downstream genes ( tgp1 + and pho1 + , respectively) by transcriptional interference, not by the formation of transient heterochromatin. We base this conclusion on our findings that: (i) tgp1 + and pho1 + expression is unaffected by loss of RNAi/heterochromatin; (ii) H3K9me2 is not associated with tgp1 + or pho1 + loci in wild-type cells; (iii) nc-tgp1 transcription declines when tgp1 + is induced (−PO 4 ); (iv) loss of the nc-tgp1 transcript allows induction of tgp1 + under normally repressive (+PO 4 ) conditions (similarly, loss of lncRNA transcription upstream induces pho1 + in repressive medium [27] , [28] ); (v) transcription of nc-tgp1 by a thiamine-repressible promoter brings tgp1 + under the control of thiamine, rather than phosphate; (vi) RNAPII and nucleosome density is increased over the tgp1 + promoter region when the repressive nc-tgp1 RNA is transcribed and (vii) the Pho7 activator binds the tgp1 + promoter region when nc-tgp1 transcription is lost. Genome-wide RNA sequencing has allowed the detection of a large number of lncRNAs in a variety of species. However, it remains unclear how many of these lncRNA are functional transcripts that act to influence gene expression and/or chromatin landscapes. Examples such as Xist RNA in mammals and roX RNAs in Drosophila represent functional transcripts that are critical for mediating dosage compensation by altering chromatin status and expression levels from sex chromosomes [47] . However, enthusiasm for lncRNA function has been somewhat dampened by reports showing that the ablation in animal models of some of the best-characterized lncRNAs (for example, HOTAIR, MALAT1, Kcnq1ot1, NEAT1) exhibited less dramatic or undetectable phenotypes [48] , [49] , [50] , [51] , [52] , [53] . Of the discrete stable lncRNAs that we deleted in fission yeast, only one ( ncRNA.1343 ) had an obvious phenotype in the growth conditions tested. Detailed analysis was required to reveal that deletion of ncRNA.1343 actually affected expression of a divergent unstable lncRNA ( nc-tgp1 ) transcribed in the opposite orientation as the annotated locus. Only after further manipulation and analyses could we conclude that the expression of nc-tgp1 interferes with the expression of tgp1 + downstream. The fact that the unstable nc-tgp1 transcript is the functional partner of the apparently non-functional stable nc-1343 RNA transcribed from the same bidirectional promoter demonstrates the importance of comprehensive analyses of ncRNAs and the consequences of their deletion. Based on our analyses. we surmise that the low level expression of nc-1343 represents transcriptional noise, resulting as a byproduct of ample nc-tgp1 transcription. The syntenic conservation of ncRNA.1343 within the Schizosaccharomyces genus [31] hints at the possibility of a conserved regulatory mechanism that involves lncRNA transcription into the promoter region of tgp1 + in related species. Thus, although genome-wide approaches can rapidly catalogue the presence and response of various lncRNAs to different conditions, much more detailed locus-specific analyses is required to pinpoint the function of each individual lncRNA with respect to cis regulation of nearby genes or trans regulation of genes at distal loci. Yeast strains, plasmids and standard techniques S. pombe strains used in this study are listed in Supplementary Table 1 . Standard methods were used for fission yeast growth, genetics and manipulations [54] . All strains were grown in Yeast extract plus supplement medium (YES), unless otherwise indicated. For phosphate starvation experiments, cells were grown to mid-log phase in YES medium, washed twice in dH 2 O, and then grown for indicated times in Pombe minimal glutamate (PMG) synthetic medium without Na 2 HPO 4 (−PO 4 ). Genetic deletions and protein tagging were carried out by lithium acetate transformation. All genetic modifications were confirmed by colony PCR. Plasmids were transformed by electroporation. Selections were performed on PMG/agar plates with according auxotrophy or on YES/agar plates with appropriate antibiotic(s) and grown at 32 °C. Serial (1:4) dilutions of equal number of cells were spotted onto YES/agar and grown at 32 °C, unless indicated otherwise. For drug-sensitivity experiments, cells were spotted onto YES/agar or PMG/agar with DMSO or TBZ (20 μg ml −1 ), HU (10 mM), caffeine (15 mM) and H 2 O 2 (1 mM). For ultraviolet-sensitivity experiments, spotted cells were ultraviolet-irradiated at 80 J m −2 with a Stratalinker UV Crosslinker and grown in the dark at 25 °C. The plasmids containing lacZ under the control of the nc-tgp1 and nc-1343 bidirectional promoter were cloned as follows. The non-coding promoter was amplified from S. pombe genomic DNA in both orientations (using lacZ_1_F/lacZ_1_R and lacZ_2_F/lacZ_2_R primer pairs; see Supplementary Table 2 ) and ligated into pREP vector containing lacZ using PstI/SalI restriction sites. To test if nc-tgp1 can repress tgp1 + in trans , the nc-tgp1 transcription unit was amplified from S. pombe genomic DNA (using nc-tgp1_SalI_F and nc-tgp1_XmaI_R primer pairs, see Supplementary Table 2 ) and ligated into pREP3x using SalI/XmaI restriction sites. Liquid assay for β-galactosidase activity Assays for β-galactosidase activity were performed as described [55] . Briefly, yeast containing vectors expressing lacZ under the control of various promoters were grown to log phase (OD 595 of ~0.5) in selective media. Cells were permeabolized by SDS/chloroform. Cell extracts were equilibrated at 30 °C for 5 min before the addition of ortho-Nitrophenyl-β-galactoside (ONPG). The reaction was stopped with Na 2 CO 3 once the solution turned yellow and elapsed time was recorded. Cell debris was spun and the OD 420 was measured. Units were calculated as follows: Units/OD=1000 × (OD 420 /Volume × Time × OD 595 ). Chromatin and RIP Cells were grown to mid-log phase at 32 °C in YES. For phosphate starvation experiments, cells in mid-log phase were washed twice in dH 2 O before being grown in PMG (−PO 4 ) for 4 h. ChIP was performed essentially as described [12] . Briefly, cells were fixed with 1% paraformaldehyde for 15 min at room temperature. Cells were lysed by bead beating (Biospec Prodcutes) and sonicated using a Bioruptor (Diagenode) sonicator at 5 °C on high for a total of 20 min (30 s ON/OFF cycles). Five microlitres of Rpb1 antibody (#2629; Cell Signaling), 2 μl GFP antibody (G10362; Life Technologies), 2 μl H3 antibody (ab1791; Abcam) and 1 μl of H3K9me2 antibody (m5.1.1; ref. 56 ) were used for IPs. RIP experiments were performed essentially as described [13] . Hisx6-TEV-Protein A-tagged Mmi1 was captured from cell lysate with IgG Dynabeads (Life Technologies). Mmi1-bound RNA was isolated by phenol-chloroform extraction, DNase treated and reverse transcribed. Quantitative analysis was performed by qPCR. RNA analysis RNA was isolated from S. pombe using RNeasy Mini- or Midi-Kits as per manufacturer’s instructions (Qiagen). For RT–qPCR experiments, first strand complementary DNA synthesis was performed on Turbo DNase (Life Technologies) treated RNA using random hexamers and Superscript III (Invitrogen) as per manufacturer’s instructions. Negative controls lacking RT were performed alongside all RT–qPCR experiments. Northern analysis of long non-coding transcripts was performed using UTP-[a 32 P]-labelled RNA probes as described [57] . Transcription start sites were mapped using the SMARTer RACE complementary DNA Amplification Kit as per manufacturer’s instructions (Clontech). Quantitative real-time PCR Primers used in this study are listed in Supplementary Table 2 . qPCR was performed using SYBR Green on a Roche Lightcycler. Data was analyzed with LightCycler 480 Software 1.5.0.39. RT–qPCR levels were calculated by normalizing product of interest to an internal reference gene ( act1 + ). Expression levels were expressed relative to levels detected in wild-type cells. ChIP enrichments were calculated as the ratio of product of interest from IP sample normalized to the corresponding input sample and expressed as ‘%IP’. Error bars represent s.e.m., resulting from at least three independent replicates. How to cite this article: Ard, R. et al . Long non-coding RNA-mediated transcriptional interference of a permease gene confers drug tolerance in fission yeast. Nat. Commun. 5:5576 doi: 10.1038/ncomms6576 (2014).